Nano-engineered electron–hole exchange interaction controls exciton dynamics in core–shell semiconductor nanocrystals A strong electron–hole exchange interaction (EI) in semiconductor nanocrystals (NCs) gives rise to a large (up to tens of meV) splitting between optically active ('bright') and optically passive ('dark') excitons. This dark–bright splitting has a significant effect on the optical properties of band-edge excitons and leads to a pronounced temperature and magnetic field dependence of radiative decay. Here we demonstrate a nanoengineering-based approach that provides control over EI while maintaining nearly constant emission energy. We show that the dark–bright splitting can be widely tuned by controlling the electron–hole spatial overlap in core–shell CdSe/CdS NCs with a variable shell width. In thick-shell samples, the EI energy reduces to <250 μeV, which yields a material that emits with a nearly constant rate over temperatures from 1.5 to 300 K and magnetic fields up to 7 T. The EI-manipulation strategies demonstrated here are general and can be applied to other nanostructures with variable electron–hole overlap. The electron–hole exchange interaction (EI) is an intrinsic property of semiconductors that impacts critical excitonic fine structure details, such as the energetic ordering of optically allowed ('bright') and forbidden ('dark') exciton states. Whereas in bulk II–VI materials exchange energies are characteristically small, just 0.13 meV for CdSe [1] , quantum-confined semiconductor nanocrystals (NCs) of the same composition exhibit much larger energies on the order of 2–20 meV [2] , [3] , [4] , [5] . Such 1–2-order-of-magnitude increases in exchange energies are significant as NC materials that exhibit large emission rates at high temperatures (radiative lifetime τ r ~10–20 ns at 300 K in CdSe NCs) become very slow emitters at low temperatures ( τ r ~1 μs at 1 K) [2] , [6] . The EI leads to this strong temperature dependence as it produces a fine structure with a lowest-energy dark exciton state and a higher-lying bright exciton state [2] . It also markedly affects other important physical properties of nanostructures, such as exciton recombination and spin dynamics [7] , [8] , coherent interdot coupling [9] and electron transfer kinetics to external quenchers [10] . The dark–bright splitting (Δ DB ), which directly relates to the EI energy, has been shown to be tunable by control of NC size from nearly 20 meV for small NCs to ~2 meV for large particles [5] . However, such size-dependent reduction of EI is accompanied by a significant change of the emission wavelength, resulting from progressively weaker quantum confinement in larger NCs. In this work, we demonstrate a means to drastically reduce EI in quasi-type II CdSe/CdS core–shell NCs [11] while preserving a nearly constant emission energy. Several reports have focused on the intrinsic effects of NC size-dependent exchange energy in II–VI NC materials [2] , [4] , [12] . Nirmal et al . established for the first time that the EI was enhanced relative to the bulk material by magnetic field-dependent studies of low-temperature time-resolved photoluminescence (trPL) and fluorescence line-narrowing (FLN) experiments [2] . Crooker et al . utilized trPL measurements as a function of temperature to determine the radiative lifetimes of both the ground-state dark exciton and the thermally accessible bright exciton state [6] . In concurrence with the FLN results of refs 2 , 3 , this work confirmed that a characteristic splitting energy dictated the relative thermal populations of dark and bright excitons in NC ensembles [13] . Importantly, it was also shown that overcoating of CdSe NCs with thin ZnS-passivating layers results in no significant change of EI or temperature-dependent photoluminescence (PL) dynamics [6] . LeThomas et al . showed that the ordering of fine structure states changes in elongated CdSe rods that exhibit differing quantum confinement effects in radial versus axial directions [14] . On elongation, the dark exciton becomes higher in energy than the bright exciton, which results in accelerated radiative recombination with reduced temperature. Here we examine heterostructured NCs comprising a CdSe core and a CdS shell of variable thickness of up to 19 CdS monolayers. These nanostructures have been a subject of recent interest owing to observations of suppressed PL intermittency ('blinking') [15] , [16] in single NC studies and suppressed biexcitonic Auger recombination [11] , [17] , [18] that leads to ultra-broad optical amplification bandwidth with record-low excitation threshold [11] and efficient multiexciton emission [18] . Reduced rates of Auger decay have also been demonstrated for other types of colloidal heteroparticles such as CdTe/CdSe [19] and CdZnSe/ZnSe [20] NCs, as well as CdSe/CdS quantum-dot/quantum-rod structures [21] . Such properties are desirable for applications ranging from optical tagging and bioimaging to telecommunications, lasing and display technology. Previous studies of CdSe/CdS NCs indicate that these systems exhibit quasi-type II electronic structure wherein the hole of an exciton is confined to the CdSe core and the comparatively light electron is delocalized over the entire core–shell nanostructure [11] , [22] . On the basis of the report of Efros et al ., [5] which indicates that enhanced wave function overlap of electrons and holes dominates the increase of EI in NCs relative to bulk, we expect that this quasi-type II motif with controlled wave function overlap presents a means to control the dark–bright splitting in these structures. The effect of electron–hole spatial separation on EI has been recently invoked to explain observations of variable spin relaxation times in core–shell CdTe/CdSe NCs [8] . However, the measurements of the EI energy as a function of electron–hole overlap, which would unequivocally demonstrate a direct relationship between these two physical quantities, are still lacking in the literature. Further, there have been no demonstrations of nanoscale systems for which the EI energy can be tuned while maintaining the same degree of quantum confinement, that is, the same emission energy. We use CdSe/CdS core–shell NCs as a model system, which allows for facile control of the electron–hole spatial separation by varying the thickness of the CdS shell. CdSe/CdS NCs can be synthesized using successive ion-layer absorption and reaction methods [15] , which allow for the fine control of the shell thickness without introducing detrimental structural defects that lead to trapping and consequent reduction of PL quantum yield. We apply three different techniques (temperature and magnetic field-dependent trPL as well as FLN measurements) to evaluate the EI energy as a function of the electron–hole overlap integral and observe a linear relationship between these two quantities. Furthermore, we demonstrate that, in this material system, the EI strength can be tuned independently of the emission energy, with the latter being controlled primarily by the size of the CdSe core. Finally, we observe several interesting peculiarities in the measured excitonic dynamics in these NCs. Specifically, highly temperature-dependent trPL, typical of CdSe NC behaviour, is detected for thin CdS shells, whereas at large shell thickness we observe nearly temperature independent lifetimes that are, furthermore, independent of magnetic fields. All of these observations can be quantitatively explained by taking into consideration temperature-dependent distribution of excitons between the 'bright' and the 'dark' fine structure states, and by using the measured EI energies. Temperature dependence of exciton dynamics Increasingly thick layers of a CdS shell were grown (from 4 to 19 monolayers) on a fixed CdSe core (radius R =1.5 nm), using methods described below [15] . 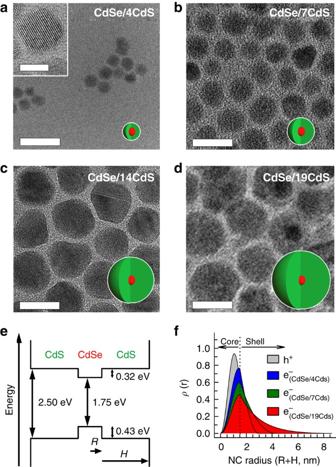Figure 1: Transmission electron microscopy images and electronic structure of CdSe/CdS NCs. CdSe/xCdS NCs with core radius,R=1.5 nm, and increasing shell thickness (a,x=4;b,x=7;c,x=14; andd,x=19 CdS monolayers, corresponding toH=1.6,H=2.8,H=5.6 andH=7.6 nm). Scale bars ina–dpanels correspond to 20 and 2 nm in the inset ofa. Schematic representations of the NCs structure are reported for each set of NCs for a fixed core radius. (e) A band alignment diagram of bulk CdSe and CdS; the band offset at the CdSe/CdS interface is not well known and in our calculations was varied from 0 to 0.32 eV (seeSupplementary Information). (f) Spatial probability distribution,ρ(r), of the hole (grey area) and electron (coloured areas) forR=1.5 nm andH=1.6 nm (blue area),H=2.8 nm (green area) andH=7.6 nm (red area);ρ(r)r2|ψe,h|2, whereψe,hare the electron (e) and the hole (h) wave functions. Representative transmission electron microscopy images of the investigated NCs are shown in Figure 1a–d . Figure 1e depicts a band alignment diagram of bulk CdSe and CdS. The spatial probability distributions, ρ ( r ), of the hole and the electron in CdSe/CdS NCs for various shell thicknesses are shown in Figure 1f (see section 'Effective mass calculations of e–h overlap and EI energies' for computational details). The electron wave function exhibits increasing leakage from the core region with increasing shell thickness, whereas the hole remains confined to the CdSe core; these behaviours result in a progressive decrease of the electron–hole spatial overlap. Figure 1: Transmission electron microscopy images and electronic structure of CdSe/CdS NCs. CdSe/ x CdS NCs with core radius, R =1.5 nm, and increasing shell thickness ( a , x =4; b , x =7; c , x =14; and d , x =19 CdS monolayers, corresponding to H =1.6, H =2.8, H =5.6 and H =7.6 nm). Scale bars in a – d panels correspond to 20 and 2 nm in the inset of a . Schematic representations of the NCs structure are reported for each set of NCs for a fixed core radius. ( e ) A band alignment diagram of bulk CdSe and CdS; the band offset at the CdSe/CdS interface is not well known and in our calculations was varied from 0 to 0.32 eV (see Supplementary Information ). ( f ) Spatial probability distribution, ρ ( r ), of the hole (grey area) and electron (coloured areas) for R =1.5 nm and H =1.6 nm (blue area), H =2.8 nm (green area) and H =7.6 nm (red area); ρ ( r ) r 2 | ψ e,h | 2 , where ψ e,h are the electron (e) and the hole (h) wave functions. Full size image For each sample, we measured both steady-state and trPL responses of drop-cast films with indicated CdS monolayer thicknesses. 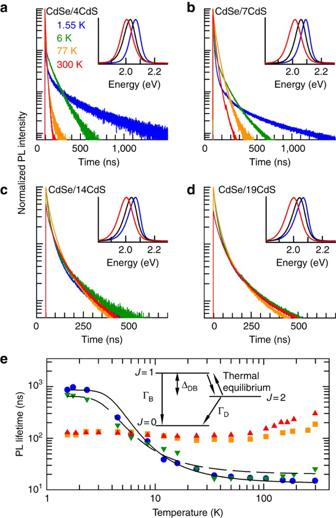Figure 2: Photoluminescence dynamics in CdSe/CdS NCs as a function of temperature. Photoluminescence (PL) decay curves measured at the emission maximum for drop-cast films of CdSe/xCdS NCs (a,x=4;b,x=7;c,x=14; andd,x=19) at the indicated temperatures (excitation energy is 3.06 eV). Steady-state PL spectra with increasing temperature (1.55 K, blue curve; 185 K, black curve and 300 K, red curve) for each sample are reported as insets in 'a–d'. (e) PL lifetimes as a function of temperature for the different CdSe/xCdS NCs (x=4, blue dots;x=7, green triangles;x=14, orange squares; andx=19, red triangles). Fits to equation (1) are reported as solid and dashed lines for CdSe/4CdS (ΔDB=1.85 meV) and CdSe/7CdS NCs (ΔDB=1.38 meV), respectively. Inset: three-level model of bright (J=1) and dark (J=2) exciton states separated by energy ΔDB. Figure 2a–d reports the PL decay curves recorded at the emission maxima for the different NCs. PL spectra at three representative temperatures ( T =1.55, 185 and 300 K) are reported as insets. The spectral position of the PL band as a function of shell thickness is roughly constant (see below and Supplementary Fig. S1 ). Moreover, both the PL band maxima and full width at half maximum for all samples behave similarly as a function of temperature regardless of the shell thickness. Figure 2: Photoluminescence dynamics in CdSe/CdS NCs as a function of temperature. Photoluminescence (PL) decay curves measured at the emission maximum for drop-cast films of CdSe/ x CdS NCs ( a , x =4; b , x =7; c , x =14; and d , x =19) at the indicated temperatures (excitation energy is 3.06 eV). Steady-state PL spectra with increasing temperature (1.55 K, blue curve; 185 K, black curve and 300 K, red curve) for each sample are reported as insets in ' a – d '. ( e ) PL lifetimes as a function of temperature for the different CdSe/ x CdS NCs ( x =4, blue dots; x =7, green triangles; x =14, orange squares; and x =19, red triangles). Fits to equation (1) are reported as solid and dashed lines for CdSe/4CdS (Δ DB =1.85 meV) and CdSe/7CdS NCs (Δ DB =1.38 meV), respectively. Inset: three-level model of bright ( J =1) and dark ( J =2) exciton states separated by energy Δ DB . Full size image Comparison of the different samples shows a prominent difference between the temperature dependence of the PL lifetimes of NCs having thin (4 and 7 monolayers) and thick CdS shells (14 and 19 monolayers). Thin CdS shell samples exhibit highly temperature-dependent PL lifetimes in similarity to previous reports for CdSe NCs with either organic or inorganic passivation [6] . At high temperatures, the dynamics are predominantly single exponential, whereas multiexponential dynamics appear at low temperature. A fast initial decay at low temperature is thought to be due to thermalization of excitons from the higher-energy bright state (net spin projection J =1) to a lower-lying J =2 dark state, or cooling of NCs as a whole due to heat exchange with the bath (matrix), followed by a much slower decay arising from recombination of dark excitons in equilibrium with the bath. With increasing temperature, the radiative lifetime becomes progressively shorter, as a result of thermal excitation of dark excitons to the bright upper exciton state [6] , [23] . Thicker-shell NCs, in contrast to the thin-shell 'typical behaviour,' exhibit nearly temperature independent dynamics (from 1.5 to 300 K). To directly compare temperature-dependent trends in exciton dynamics of different samples, we fit trPL traces to double exponential decay and assign a slower time constant to radiative lifetime, τ r (see Methods and Supplementary Information for details of this procedure and verifications of its validity). For traces measured at T <10 K for thin-shell samples, we disregard a fast initial signal drop as it is not due to recombination but rather by thermalization; this approach allows us to avoid non-recombination-related contributions to derived time constants and is common in the analysis of low-temperature excitonic dynamics in CdSe NCs [2] , [6] . Figure 2e reports the evolution of τ r with temperature for four samples. For thin-shell NCs, τ r is 860 ns at temperatures below 3 K and undergoes a 2-order-of-magnitude decrease at higher temperatures. In agreement with previous literature, we ascribe this effect to the thermal activation between the dark and the bright exciton states [6] . By assuming a Boltzmann distribution of excitons between these two states, we can model the transition between the slow and fast decay regimes in a simple three-level scheme (inset of Fig. 2e ), by expressing the radiative decay rate as: where Γ 0D and Γ 0B are the radiative decay rates of the dark and bright states [6] . The above model exhibits excellent agreement with the experimental data for CdSe NCs having four and seven CdS monolayer shells, yielding Δ DB =1.85 meV and Δ DB =1.38 meV for the two samples, respectively. NCs with 14- and 19 CdS monolayer shells show only very weak variation with temperature, from ~116 ns at 1.5 K to 200–300 ns at 300 K. These almost temperature independent radiative lifetimes of the thick CdS shell samples suggest that the dark–bright energy splitting has become significantly smaller with respect to conventional CdSe NCs. Fluorescence line-narrowing experiments To directly measure the dark–bright energy splitting in thick-shell samples, we perform FLN measurements. 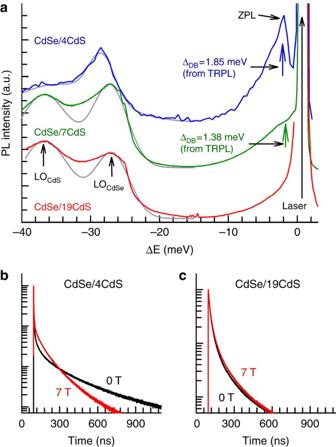Figure 3: Fluorescence line-narrowing spectra and magnetic field dependence of the emission dynamics. (a) Fluorescence line-narrowing (FLN) spectra at 1.55 K for CdSe/4CdS (blue curve, excitation energyEEX=2.101 eV), CdSe/7CdS (green curve,EEX=2.138 eV) and CdSe/19CdS NCs (red curve,EEX=2.138 eV). A portion of the excitation laser is included for reference and set to zero for direct comparison between the different NCs. The values for the Stokes shift, ΔDB, between the excitation pump and the zero-phonon (ZP) line extracted from the Boltzmann fit of the temperature-dependent fluorescence lifetimes (τR(T)) are indicated by arrows. Gaussian fits of the CdSe and CdS LO phonon bands are shown by grey curves. The deviations of the experimental spectra from simple double-Gaussian fits are likely due to contributions from surface phonons that were not included in the fitting procedure. PL decay curves at the emission maxima (excitation energy is 3.06 eV) at 0 T (black curve) and 7 T (red curve) for (b) CdSe/4CdS and (c) CdSe/19CdS NCs. Figure 3a shows FLN spectra at 1.55 K of the same NC samples as in Figure 2 , excited on the red edge of the lowest-energy 1S absorption feature, which selects only the lowest band-gap NCs in the ensemble. Whereas photoexcitation of the entire NC ensemble produces a broad Gaussian PL feature that arises because of NC-size distribution (insets of Fig. 2a,d ), FLN spectra exhibit several distinct, relatively narrow peaks. In qualitative agreement with previous studies of CdSe NCs [2] , [3] , [24] , the FLN spectrum of the CdSe/4CdS NC sample shows a pronounced zero-phonon (ZP) line that is red-shifted by ~2 meV with respect to the photoexcitation energy corresponding to the J =1 (bright) exciton. This ZP feature results from radiative recombination of the nominally forbidden dark J =2 state [2] , [3] . In addition, we detect two lower-energy features separated from the ZP line by 25 and 35 meV, which are due to phonon-assisted recombination of a dark exciton involving CdSe and CdS phonons, respectively. Figure 3: Fluorescence line-narrowing spectra and magnetic field dependence of the emission dynamics. ( a ) Fluorescence line-narrowing (FLN) spectra at 1.55 K for CdSe/4CdS (blue curve, excitation energy E EX =2.101 eV), CdSe/7CdS (green curve, E EX =2.138 eV) and CdSe/19CdS NCs (red curve, E EX =2.138 eV). A portion of the excitation laser is included for reference and set to zero for direct comparison between the different NCs. The values for the Stokes shift, Δ DB , between the excitation pump and the zero-phonon (ZP) line extracted from the Boltzmann fit of the temperature-dependent fluorescence lifetimes ( τ R ( T )) are indicated by arrows. Gaussian fits of the CdSe and CdS LO phonon bands are shown by grey curves. The deviations of the experimental spectra from simple double-Gaussian fits are likely due to contributions from surface phonons that were not included in the fitting procedure. PL decay curves at the emission maxima (excitation energy is 3.06 eV) at 0 T (black curve) and 7 T (red curve) for ( b ) CdSe/4CdS and ( c ) CdSe/19CdS NCs. Full size image On increasing the shell thickness, notable changes appear in the FLN spectra. Most importantly, the ZP feature becomes less pronounced with increasing CdS shell thickness and is essentially undetectable for the CdSe/19CdS NCs sample. This trend is consistent with a progressive reduction in the spacing between the J =2 and J =1 excitons until it becomes unresolvable, given limited instrumental spectral resolution. The dark–bright energy splitting extracted from the analysis of the temperature-dependent PL lifetimes of the four-monolayer sample (1.85 meV) is in good agreement with the Stokes shift between the laser pump and the ZP line observed in the FLN spectrum (1.87 meV). As for samples with a thicker shell, the ZP line is not directly resolvable, we use the positions of the phonon replicas to derive the dark–bright exciton splitting. Specifically, we notice that the energy shift of the phonon-assisted features with respect to the excitation laser is progressively reduced with increasing shell thickness as expected for the situation in which the ZP emission line shifts towards the laser line. The spectral position of the phonon features in the FLN spectra can therefore be used to probe the dark–bright splitting for thick-shell NCs. To do so, we use CdSe/4CdS NCs as a reference to measure the energy shift between the ZP line and the first phonon feature (LO CdSe ) and subtract its value from the energy of the same LO CdSe feature for thicker-shell NCs, which we obtained by a Gaussian fit of the respective FLN peaks (grey lines in Fig. 3a ). For CdSe/19CdS NCs, this procedure produces Δ DB =0.27 meV, which is about 1-order-of-magnitude smaller than that for CdSe/4CdS NCs and is in good agreement with the EI energy obtained by analysis of the PL dynamics, as shown later in this paper. Therefore, both trPL and FLN results suggest the progressive reduction of the dark–bright energy splitting for increasing shell thickness. Exciton recombination dynamics under applied magnetic fields To further confirm this controlled reduction of the EI, we perform trPL under applied magnetic fields (0–7 T). Magnetic fields both Zeeman split and quantum mechanically mix proximal exciton states. In previous low-temperature trPL measurements of CdSe NCs, magnetic fields were found to accelerate radiative rates owing to field-induced mixing of bright exciton character into the dark exciton [2] , [25] . Figure 3b,c shows magnetic field-dependent trPL data for 4- and 19-shell NC samples. The magnetic field notably decreases the radiative lifetime for the four-shell sample, but does not induce any discernable changes in the decay rate for the 19-shell sample. These results again suggest that indeed the EI approaches zero in samples with a large CdS shell thickness. Effective mass calculations of e–h overlap and EI energies Previous studies of CdSe NCs indicate a strong dependence of dark–bright exciton splitting on emission wavelength, which reflects a direct dependence of EI on NC size [2] , [6] . The NC-size arguments, however, are unlikely to explain the observed changes in Δ DB in our core–shell samples. Although the overall size of the NC is increased with increasing shell thickness ( H ), the emission wavelength in these samples is almost insensitive to this parameter. 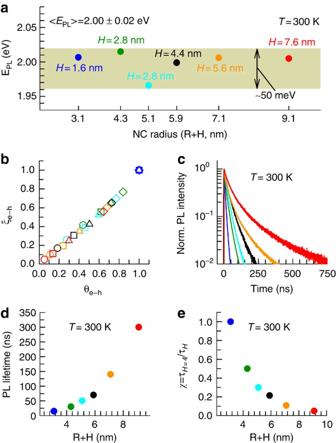Figure 4: Room-temperature emission energies (EPL), radiative lifetimes and calculated exchange interaction terms (ξe−h). (a) Peak emission energy as a function of the total NC size (excitation energy is 3.06 eV). All NCs have the same CdSe core radiusR=1.5 nm. Different thicknesses of the CdS shell (H) correspond to different colours that are used to colour-code data in four other panels of the figure (H=1.6 nm, blue;H=2.8 nm, green;H=3.6 nm, cyan;H=4.4 nm, black;H=5.6 nm, orange;H=7.6 nm, red). (b) Exchange interaction term,ξe−h, as a function of electron–hole overlap integral (θe−h) calculated according to refs11and22for different values for the conduction-band energy offset at the CdSe/CdS interface: ΔEe=0 (circles), 0.1 eV (squares), 0.2 eV (triangles) and 0.32 eV (diamonds, seeSupplementary Information). Bothθe−hand ξe−hare normalized to the respective values obtained for CdSe/4CdS (H=1.6 nm). Experimental results for (c) PL dynamics, (d) radiative lifetimes and (e)χ=as a function of total NC size. For example, as evident from Figure 4a , both the thinnest and the thickest shell samples studied here emit at the same energy of 2.01 eV ( T =300 K), whereas in other samples the emission energy is within ±25 meV of this value. These observations strongly suggest that the effective exciton size in our samples is not significantly dependent on the overall NC dimensions but is defined primarily by the core size (see Supplementary Information ). Figure 4: Room-temperature emission energies ( E PL ), radiative lifetimes and calculated exchange interaction terms ( ξ e−h ). ( a ) Peak emission energy as a function of the total NC size (excitation energy is 3.06 eV). All NCs have the same CdSe core radius R =1.5 nm. Different thicknesses of the CdS shell ( H ) correspond to different colours that are used to colour-code data in four other panels of the figure ( H =1.6 nm, blue; H =2.8 nm, green; H =3.6 nm, cyan; H =4.4 nm, black; H =5.6 nm, orange; H =7.6 nm, red). ( b ) Exchange interaction term, ξ e−h , as a function of electron–hole overlap integral ( θ e−h ) calculated according to refs 11 and 22 for different values for the conduction-band energy offset at the CdSe/CdS interface: Δ E e =0 (circles), 0.1 eV (squares), 0.2 eV (triangles) and 0.32 eV (diamonds, see Supplementary Information ). Both θ e−h and ξ e−h are normalized to the respective values obtained for CdSe/4CdS ( H =1.6 nm). Experimental results for ( c ) PL dynamics, ( d ) radiative lifetimes and ( e ) χ = as a function of total NC size. Full size image In addition to the effective exciton size, the e–h exchange coupling depends critically on the spatial overlap between the electron and the hole. Evaluation of this overlap is especially important in hetero-NCs in which the spatial distributions of electrons and holes can be very different. To evaluate the effect of electron–hole spatial overlap on EI, we use a standard approach based on the effective mass approximation (EMA). This approximation has been successfully applied previously to describing electronic spectra in CdSe NCs (including the fine structure excitonic splitting) for a wide range of radii down to values of 1 nm (refs 2 , 3 , 4 ). More recently, EMA models were successfully used to calculate electronic structures and exciton–exciton interactions in core–shell NCs of compositions such as CdS/ZnSe [22] , [26] , ZnSe/CdSe [27] , [28] , CdSe/ZnS [29] , [30] , CdTe/CdS [31] and PbSe/CdSe [32] . In EMA models, electronic wave functions are described in terms of a product of the Bloch function and the envelope wave function (ψ e and ψ h are the electron and hole envelope functions, respectively). In the case of our nearly spherical NCs, the exchange coupling is dominated by the short-range interaction, which is directly proportional to the quantity , refs 33 , 34 . To calculate ξ e−h , we use the two-band EMA formalism from refs 11 and 22 . This formalism does not account for band-mixing effects. However, it still allows us to capture essential trends associated with variations of shell thickness because in CdSe/CdS NCs, changes in H affect ξ e−h primarily through changes in ψ e , which is not strongly influenced by band mixing. Specifically, in CdSe/CdS NCs, the increase in shell thickness leads to increased leakage of the electron wave function into the shell region without significantly affecting the spatial distribution of the hole wave function, which remains confined to the core ( Fig. 1f ). These behaviours lead to a reduction of the electron–hole spatial overlap, which, within the EMA, can be quantitatively characterized by the overlap integral involving envelope wave functions: . In our modelling, we assume a sharp, step-like potential at the CdSe/CdS interface. However, we would like to point out that very recent FLN studies of CdSe/CdS nanostructures suggest the formation of a thin alloyed layer (~1–2 monolayers) due to a small degree of Se/S intermixing at the core–shell interface [35] . This interfacial alloying or 'smoothing' does have profound implications for Auger recombination dynamics that are very sensitive to the abruptness of the interface [36] . However, this slight Se/S alloying at the core–shell boundary does not alter the depth or the mean width of the confinement potential, and therefore should only minimally affect the spatial extent and the overlap of the electron and the hole wave functions. Interestingly, our calculations indicate that for CdSe/CdS NCs, changes in ξ e−h with increasing H are in close correspondence with the changes in θ e−h , which results in almost perfectly linear dependence of ξ e−h on θ e−h ( Fig. 4b ). This result strongly suggests that, in these nanostructures, Δ DB is directly proportional to θ e−h : Δ DB =Δ 0 θ e−h , where Δ 0 is the EI splitting in the case in which the electron–hole overlap is unity. To experimentally evaluate the changes in the electron–hole overlap with increasing H , we analyse room-temperature radiative lifetimes ( Fig. 4c,d ). At room temperature, when k B T ≫ Δ DB , radiative decay occurs primarily through the bright exciton state, which accommodates half of the exciton population. In this case, the change in shell thickness does not affect the exciton distribution between the bright and the dark states, and the PL decay rate varies solely because of the change in the spatial distributions of electron and hole wave functions. To characterize this change, we introduce a dimensionless parameter χ , which we calculate by normalizing the PL decay rate (Γ=1/ τ r ) measured for different samples by the rate observed for the thinnest-shell (4 CdS monolayers) NCs ( τ r ≈15 ns). The data derived in this way ( Fig. 4e ) indicate that χ progressively decreases with increasing H and is ~0.05 in the case of the 19 CdS monolayer sample. This drop in χ is due to a progressive increase in the mismatch between the volumes occupied by the electron and the hole in the course of expansion of the electron wave function into the shell region. As within the EMA, the radiative decay rate is directly proportional to θ e−h (Γ=1/ τ r θ e−h ) (refs 5 , 34 ), the measured changes in χ should reproduce the variations in θ e−h : θ e−h = aχ , where a is a proportionality constant. To incorporate the effect of electron–hole overlap into equation (1), we assume the validity of EMA, which allows us to express the radiative decay rates of the bright and the dark excitons as Γ D = θ e−h Γ 0D and Γ B = θ e−h Γ 0B (refs 5 , 37 ). On the basis of the results of our modelling ( Fig. 4b ), we also assume a linear scaling of the dark–bright energy splitting with θ e−h . These assumptions lead to the following generalized version of equation (1), which would apply to samples with a nonunity electron–hole overlap integral: In this generalized form, equation (2) accounts for the effect of varying electron–hole overlap on both the emission rate of a given exciton state and the distribution of exciton population between the bright and the dark levels. To verify the validity of our model, we use it to analyse the effect of shell thickness on low-temperature PL lifetimes. 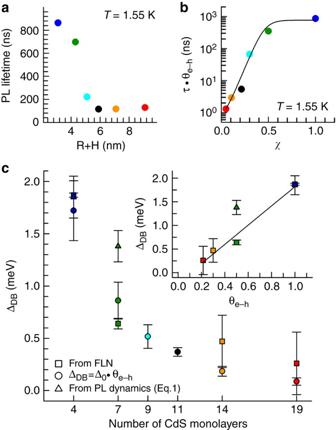Figure 5: Analysis of PL lifetimes using a variable-EI energy model. (a) Measured radiative lifetimes at 1.55 K for increasing shell thickness. All NCs have the same CdSe core radiusR=1.5 nm. Different thicknesses of the CdS shell (H) correspond to different colours that are used to colour-code data in two other panels of the figure and in the inset of 'c' (H=1.6 nm, blue;H=2.8 nm, green;H=3.6 nm, cyan;H=4.4 nm, black;H=5.6 nm, orange;H=7.6 nm, red). (b) Same as in 'a' but as a product ofτrandχplotted versusχ(χis extracted from room-temperature PL dynamics using the relationshipχ=). A fit ofτr·χto equation (2) is shown by the solid line. (c) Dark–bright energy splitting, ΔDB, as a function of shell thickness (expressed in terms of the number of CdS monolayers) extracted from the analysis of the PL dynamics and FLN spectra. A very good agreement is observed between the ΔDBvalues obtained with the different methods. The inset shows the measured values of ΔDBas a function of the measured electron-hole overlap integral (θe−h) for increasing shell thickness. These data can be fitted closely using a linear relationship between ΔDBandθe−h(line). In Figure 5a , we plot τ r measured at 1.5 K as a function of NC total radius ( r = R + H ). In contrast to room-temperature observations in which PL lifetime increases with r , the low-temperature data indicate a different trend—a significant, almost an order-of-magnitude decrease in τ r . This trend is opposite to one expected from a progressive reduction of the electron–hole overlap and is a direct result of decreasing EI energy that leads to increased occupancy of the bright excitonic state. Figure 5: Analysis of PL lifetimes using a variable-EI energy model. ( a ) Measured radiative lifetimes at 1.55 K for increasing shell thickness. All NCs have the same CdSe core radius R =1.5 nm. Different thicknesses of the CdS shell ( H ) correspond to different colours that are used to colour-code data in two other panels of the figure and in the inset of ' c ' ( H =1.6 nm, blue; H =2.8 nm, green; H =3.6 nm, cyan; H =4.4 nm, black; H =5.6 nm, orange; H =7.6 nm, red). ( b ) Same as in ' a ' but as a product of τ r and χ plotted versus χ ( χ is extracted from room-temperature PL dynamics using the relationship χ = ). A fit of τ r · χ to equation (2) is shown by the solid line. ( c ) Dark–bright energy splitting, Δ DB , as a function of shell thickness (expressed in terms of the number of CdS monolayers) extracted from the analysis of the PL dynamics and FLN spectra. A very good agreement is observed between the Δ DB values obtained with the different methods. The inset shows the measured values of Δ DB as a function of the measured electron-hole overlap integral ( θ e−h ) for increasing shell thickness. These data can be fitted closely using a linear relationship between Δ DB and θ e−h (line). Full size image To further analyse the data, in Figure 5b we present them in terms of the product of the measured radiative decay time and χ plotted as a function of χ . According to equation (2), such a representation allows one to separate the contribution due to variable EI energy from that due to the direct effect of electron–hole overlap on Γ D and Γ B rates. Using this plot, we immediately see that changes in EI alone would lead to more than a 2-order-of-magnitude change in the PL decay constant. The measured changes in τ r , however, are weaker because the effect of the variable EI energy is partially compensated by reduction of bright- and dark-exciton decay rates produced by reduced electron–hole overlap. Finally, we analyse the data set in Figure 5b using equation (2). Specifically, equation (2) can closely reproduce a complete set of experimental data for six different core–shell samples (line in Fig. 5b ) using Δ 0 and a as adjustable parameters. The Δ 0 value produced by this fit is ~1.6 meV, which is close to the dark–bright exciton splitting of 1.5 meV measured by FLN for standard CdSe NCs emitting at a similar wavelength [3] . On the basis of the fit, a =1.1, which indicates that the experimental values of χ provide a close measure of θ e−h . An excellent agreement between the experimental results and the model described by equation (2) provides strong evidence that observed changes in EI energy are primarily due to changes in electron–hole spatial overlap but not due to changes in the overall NC size. In Figure 5c , we summarize the dark–bright splitting energies obtained by the three different approaches: direct analysis of the temperature dependence of the PL dynamics by equation (1) (thin-shell samples), analysis of the FLN spectra (that is, by direct measure of the position of the ZP feature for CdSe/4CdS NCs and by the analysis of the position of the LO CdSe peak for samples with shells containing 7–19 monolayers of CdS), and calculations using expression Δ DB =Δ 0 θ e−h (all samples), where Δ 0 is determined from fitting the low-temperature PL lifetimes by equation (2) ( Fig. 5b ) and θ e−h is derived from room-temperature lifetimes ( Fig. 4e ). The data obtained by all of these methods are in good agreement and indicate a systematic decrease in the energy of dark–bright exciton splitting with increasing shell thickness. Furthermore, the fact that the result of direct experimental measurements of PL lifetimes are closely described assuming a linear scaling of Δ DB with θ e−h indicates that the demonstrated tunability of EI energy is enabled by varying electron–hole overlap, which in CdSe/CdS NCs can be controlled by tuning the CdS shell width. A linear relationship between Δ DB and θ e−h is also evident from the plot in the inset of Figure 5c , in which we show the values of a dark–bright splitting derived from FLN (squares) and temperature-dependent PL dynamics (triangles) as a function of electron–hole overlap obtained from room-temperature PL decay rates ( Fig. 4e ). In conclusion, we have demonstrated that by increasing the thickness of a CdS shell in core–shell CdSe/CdS NCs, we can tune the EI energy from ~1.8 to ~0.1 meV. The measured radiative lifetimes as a function of shell width exhibit two opposite trends at room and cryogenic temperatures. The room-temperature time increases with H , as expected from the reduced electron–hole overlap due to increasing leakage of the electron wave function into the shell region. The low-temperature PL lifetime, instead, rapidly decreases with H , which is a direct consequence of reducing EI energy, which leads to increased occupancy of the bright exciton level. The direct correlation between evolutions of θ e−h with H (derived from room-temperature measurements) and the dark–bright splitting (obtained from FLN studies and temperature-dependent PL dynamics) strongly suggests that, in these core–shell NCs, the EI energy is directly proportional to the electron–hole overlap integral. Importantly, this tunability is achieved for a nearly constant emission energy, which provides a new tool for controlling excitonic dynamics including absolute recombination time scales and temperature and magnetic field dependences (enabling, for example, selection between strong versus weak dependence on T or B ) separately from the confinement energy. Nanocrystal synthesis and sample preparation Colloidal core/shell CdSe/CdS NCs were produced based on successive ion-layer absorption and reaction methods as reported previously [15] . The NCs were then diluted in hexane and drop-casted onto quartz substrates. Temperature and magnetic field-dependent trPL The samples were mounted in the variable temperature insert (1.5–300 K) of a 7-T split-coil superconducting magnet with direct optical access. Steady-state and trPL measurements were conducted by exciting at 3.06 eV (405 nm) with a pulsed diode laser (repetition rate 250 KHz, pulse duration ~40 ps) and collecting the emitted light with an optical fibre coupled to a monochromator, a multichannel plate detector and time-correlated single-photon counting electronics (time resolution ~200 ps). Very low excitation fluence (peak power ~2×10 15 photons pulse −1 cm −2 ) was used to avoid multiexciton excitation. Neither 10× higher nor lower laser fluence affected the results. Fluorescence line-narrowing experiments For FLN measurements, a spectrally narrow photoexcitation source (<0.2 nm FWHM) was produced by coupling the output of an 800-nm Ti:sapphire oscillator (70 mW, 80 MHz, 100 fs) into a photonic crystal-fibre white-light continuum generator, which was filtered with a 1/3 m monochromator. The emitted PL photons were collected, fibre coupled into a 1/2 m spectrograph and detected with a liquid nitrogen-cooled charged coupled device. Derivation of radiative lifetimes Measurement of trPL at multiple emission wavelengths indicated a lack of energy transfer for all NC film samples presented. PL traces were analysed using a double exponential fit, which produced two time constants τ 1 and τ 2 and two amplitudes A 1 and A 2 (as mentioned in the main text, for thin-shell samples, we analysed the low-temperature traces disregarding the fast initial drop due to thermalization). We further used the slower time constant τ 2 as a measure of a radiative lifetime, τ r = τ 2 , assuming that initial faster decay is also contributed by non-radiative processes. This 'biexponential' (or often multiexponential) behaviour is common in NC ensemble measurements and arises from coexistence of well-passivated NCs with dynamics dominated by radiative decay and poorly passivated particles, in which carrier recombination is also contributed by non-radiative processes involving surface or interfacial (in the case of core–shell structures) defects. The validity of assigning a slow constant to purely radiative decay is indicated by the following arguments. First, the same samples prepared as solutions exhibited almost a single exponential decay with a constant, which was nearly identical (within 10%) to τ 2 derived from NC film measurements. Further, in the case of biexponential PL decay with τ 2 = τ r , the emission quantum yield ( q ) is given by q =[ A 1 ( τ 1 / τ 2 ) + A 2 ]( A 1 + A 2 ) −1 . We used this expression to calculate room-temperature quantum yields for our core–shell NCs based on measured dynamics and then compared them with relative quantum yields measured by normalizing spectrally integrated steady-state PL by sample absorbitivity for constant excitation intensity. The observed remarkable agreement (within 15%) between the two data sets confirms the assignment of the τ 2 time constant to radiative decay. More details on extraction of radiative lifetimes from measured PL dynamics can be found in Supplementary Information . How to cite this article: Brovelli, S. et al . Nanoengineered electron–hole exchange interaction controls exciton dynamics in core–shell semiconductor nanocrystals. Nat. Commun. 2:280 doi: 10.1038/ncomms1281 (2011).